Homo-coupling of terminal alkynes on a noble metal surface The covalent linking of acetylenes presents an important route for the fabrication of novel carbon-based scaffolds and two-dimensional materials distinct from graphene. To date few attempts have been reported to implement this strategy at well-defined interfaces or monolayer templates. Here we demonstrate through real space direct visualization and manipulation in combination with X-ray photoelectron spectroscopy and density functional theory calculations the Ag surface-mediated terminal alkyne C sp −H bond activation and concomitant homo-coupling in a process formally reminiscent of the classical Glaser–Hay type reaction. The alkyne homo-coupling takes place on the Ag(111) noble metal surface in ultrahigh vacuum under soft conditions in the absence of conventionally used transition metal catalysts and with volatile H 2 as the only by-product. With the employed multitopic ethynyl species, we demonstrate a hierarchic reaction pathway that affords discrete compounds or polymeric networks featuring a conjugated backbone. This presents a new approach towards on-surface covalent chemistry and the realization of two-dimensional carbon-rich or all-carbon polymers. The classic route to covalent linking of acetylenes is the oxidative coupling reaction catalysed by copper ions in solution, with the initial key achievements reaching back to distant times [1] , [2] , [3] , [4] , [5] . Today, acetylenic coupling is recognized as a versatile ingredient for the rational design of carbon scaffolds and networks [6] , [7] , [8] . This procedure is notably promising for controlled fabrication of novel two-dimensional (2D) materials with carbon–carbon bonding distinct from graphene, showing emerging properties of fundamental and technological interest [8] , [9] , [10] . Thus, it is a timely issue to explore acetylenic coupling at interfaces, and recent studies using a sequential protocol with monolayer self-assembly followed by a crosslinking step provided encouraging results [11] . Pursuing a different vein, there is the prospective research domain dealing with on-surface covalent reactions under ultrahigh vacuum (UHV) conditions on clean metal surfaces to realize novel functional nano-architectures and networks [12] , [13] , [14] , [15] , [16] , [17] , [18] , [19] . However, many of the employed protocols imply appreciable activation barriers or rely on the enabling character of a set of leaving groups. For instance, interfacial Ullmann reactions can generate adsorbed halogens and thus entail the drawback of spurious by-products coexisting with the target structures [13] , [15] . Accordingly, processes with milder reaction conditions avoiding at the same time the release of contaminations are needed. The surface confinement can moreover promote unique reaction pathways. These have been nicely exemplified by cyclodehydrogenation processes on Cu(111) for tailored nanographenes [19] , or site-specific linear alkane polymerization on an Au(110) facet [20] . A recent related report reveals the prominent role of a noble metal substrate in the catalytic course of a C−C Sonogashira coupling reaction elucidating its heterogenic nature [21] . Here we demonstrate using scanning tunnelling microscopy (STM) measurements and density functional theory (DFT) calculations the Ag-mediated terminal alkyne C sp −H bond activation and concomitant homo-coupling in a surface-assisted process. The pertaining C−C covalent bond formation ( Fig. 1a ) is formally reminiscent of the so-called Glaser–Hay type coupling [1] , [4] , while simultaneously presenting a new approach towards silver-acetylide chemistry [22] , [23] . The alkyne homo-coupling takes place on the Ag(111) noble metal surface in UHV under soft conditions with volatile H 2 as the only by-product. The hierarchic reaction pathway affords discrete compounds or polymeric networks with a conjugated backbone. The mild thermal activation required, the high yields and the obtained selectivity reveal that this process belongs to a different class as the well-known alkyne C−C coupling reactions on transition metal surfaces targeting small aromatic compounds [24] . Our strategy combines the versatility and promise of acetylenic coupling in solution or bulk environments with the high prospects associated with on-surface covalent engineering of low-dimensional nano-architectures. The presently introduced C−C coupling scheme thus bears significant potential for the preparation of novel 1D or 2D materials and molecular devices, notably including carbon-pure scaffolds and compounds. 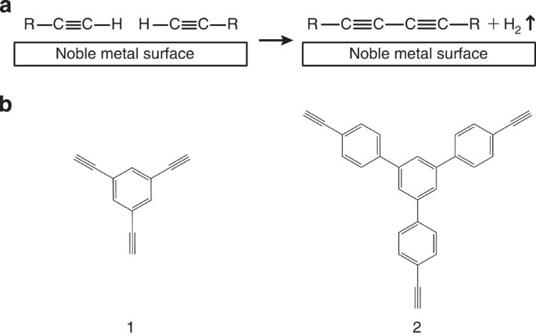Figure 1: Reaction scheme and employed molecules. (a) Surface-assisted homo-coupling reaction. (b) Terminal alkyne modules: 1,3,5-triethynyl-benzene1(TEB); 1,3,5-tris-(4-ethynylphenyl)benzene2(Ext-TEB). Figure 1: Reaction scheme and employed molecules. ( a ) Surface-assisted homo-coupling reaction. ( b ) Terminal alkyne modules: 1,3,5-triethynyl-benzene 1 (TEB); 1,3,5-tris-(4-ethynylphenyl)benzene 2 (Ext-TEB). Full size image Surface-assisted covalent dimerization of TEB modules Compound 1 molecules (1,3,5-triethynyl-benzene, named TEB, cf. Fig. 1b ) were initially deposited onto the Ag(111) surface held at 170 K, which results in self-assembled large islands with a long-range periodic structure ( Fig. 2a ). Thus, the translational and rotational motion of molecules is ensured on the poorly reactive Ag surface, which is a prerequisite for ordering and further reaction processes [25] . Within the dense-packed islands individual molecules lie flat on the surface, which is typical for benzene derivatives on noble metals, and appear as triangular protrusions (bright), consistent with the size and symmetry of the intact species. 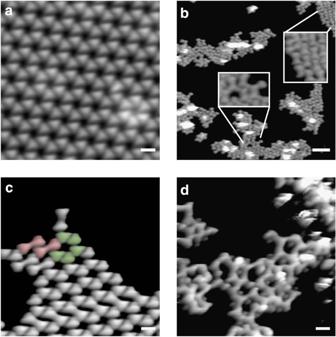Figure 2: STM topographic images of TEB molecules and reaction products on Ag(111). (a) Dense-packed phase formed by single molecules, deposited at a substrate temperature of 170 K. (b) Overview image with islands of TEB dimers, formed under a high flux on the substrate at a temperature of 330 K. The insets highlight a dimer array (upper right) and oligomeric structures (centre). (c) Area with coexisting single molecules (green) and dimeric compounds (red). (d) Oligomerization induced by annealing a dimer-dominated sample to 370 K. The scale bars ina,candddenote 10 Å, and inb50 Å. Figure 2: STM topographic images of TEB molecules and reaction products on Ag(111). ( a ) Dense-packed phase formed by single molecules, deposited at a substrate temperature of 170 K. ( b ) Overview image with islands of TEB dimers, formed under a high flux on the substrate at a temperature of 330 K. The insets highlight a dimer array (upper right) and oligomeric structures (centre). ( c ) Area with coexisting single molecules (green) and dimeric compounds (red). ( d ) Oligomerization induced by annealing a dimer-dominated sample to 370 K. The scale bars in a , c and d denote 10 Å, and in b 50 Å. Full size image Following standard procedures, the first attempt was to thermally trigger a chemical reaction by sample annealing. However, heating the surface with the adsorbed organic layer to room temperature considerably reduces the coverage of TEB molecules without inducing any morphology change in the STM appearance. Thermal annealing up to 330 K essentially restores the pristine surface free of TEB species, that is, the desorption temperature is lower than that needed to activate a reaction. Thus, we exposed the substrate kept at 330 K to a high molecular flux (partial pressure ~10 −8 mbar) to induce chemical transformation in the transient adsorption regime. Indeed, this procedure generated distinct novel surface features. The STM image depicted in Fig. 2b reveals irregular islands mainly consisting of pairwise arranged triangles connected by a waist (grey, upper right inset), designated as dimers. Only scarcely do the islands incorporate extended, interconnected arrangements (centre inset). Close inspection also reveals some features (white) ascribed to impurities of unknown nature resulting from the limited quality of the powder used for evaporation. The potential (catalytic) role of these impurities in the resulting topography is excluded in conjunction with experiments presented later. We attribute the very different appearance of the layer to the prevailing dimers recognized as novel compounds formed on the surface. For a direct comparison of individual TEB units with the dimer species we prepared a sample as described above, but additionally maintained the exposure to the molecular beam while cooling down. As a result both monomers and dimers coexist on the surface and can be imaged with exactly the same tip and scanning parameters (cf. Fig. 2c ). Monomers (highlighted in green) are clearly discernable and their assembly is locally similar to that in the supramolecular layer. By comparison, the appearance of the dimer (highlighted in red) is consistent with the size of two TEB molecules being connected by a 1,3-butadiyne group resulting from the homo-coupling of two terminal alkynes. The results suggest that under appropriate conditions the monomers can be linked by a self-limiting surface-assisted reaction favouring a high yield of dimeric products, whereby the formation of oligomers is inhibited. In fact, a statistical analysis of the sample displayed in Fig. 2b shows that approximately three quarters of the originally monomeric compound were successfully dimerized. Due to the increased surface bonding of the dimers, it is now possible to induce further changes at higher temperatures. The data in Fig. 2d evidence a drastic transformation of the dimer-dominated sample ( Fig. 2b ) upon tempering at 370 K for 10 min. Although the observed structures are rather irregular, they definitely must comprise multiple interconnections between the original TEB constituents, which can hardly be identified in the network arrangement due to the small size of the monomer unit. Covalent nature of the TEB dimer Next we address the nature of the dimeric TEB compounds by DFT simulations. We need to consider that the dimer formation proceeds under conditions where substrate step fluctuations occur and silver adatoms exist on the surface. This might interfere with the surface-assisted reaction and potentially afford organometallic Ag bis -acetylide complexes, similar to related scenarios on Cu surfaces [26] , [27] , [28] . The covalently bonded dimer was relaxed on the Ag(111) surface and an STM image simulation was carried out with the equilibrium structure ( Fig. 3a and Supplementary Fig. S1a ). The calculated image shows a smooth connexion between the two TEB moieties, which has an apparent height slightly lower than the two benzene rings. For comparison, the Ag bis -acetylide complex, further referred to as organometallic dimer, would exhibit a characteristic substructure in the connecting waist originating from the metal centre (cf. Supplementary Fig. S1b ) and furthermore its length exceeds that of the covalent dimer. The simulated STM image of a covalently bonded dimer ( Fig. 3a ) and the experimental data of a dimer ( Fig. 3b ) are rendered with the same colour code. The characteristic outline, the smooth connexion via the thinner waist, as well as the slightly brighter benzene rings compared with the waist, all agree well with the simulation. We furthermore analysed the small regular dimer patch depicted in Fig. 3c . With the model of the covalent dimer as obtained by the DFT calculations superimposed on the dimer array a very good agreement is found. The unit cell ( a =14.5 Å, b =10.2 Å, α =88.0°, β =25.0°) was determined with <0.3 Å precision (typical error<2%). Because of the extension of covalent versus organometallic dimers differs by 2.5 Å, the latter cannot be reconciled with the unit cell size ( Supplementary Fig. S1d ). Moreover, STM molecular manipulation experiments were employed to assess the stability of the connexion between the two TEB moieties of the dimer ( Supplementary Fig. S2 ). Whereas monomers can be removed from islands of the dense-packed phase without affecting the order of neighbouring molecules ( Supplementary Fig. S2a,b ), the TEB dimer could only be translated as a rigid unit under similar conditions ( Supplementary Fig. S2c,d ). 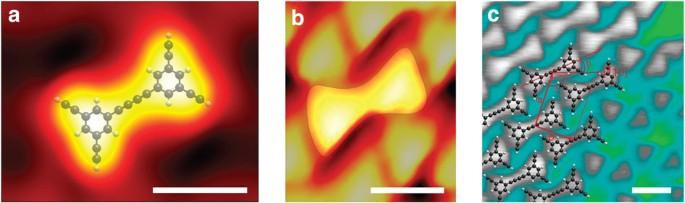Figure 3: DFT simulations and comparison with STM observations. (a) Simulated STM image of the covalent dimer on a Ag(111) slab (U=−0.6 V) with its carbon backbone. (b) High-resolution STM image of a dimer (U=−0.57 V,I=0.1 nA). (c) STM image of an ordered dimer patch superimposed with the calculated dimer structure (U=0.1 V,I=0.1 nA). All scale bars denote 10 Å. Figure 3: DFT simulations and comparison with STM observations. ( a ) Simulated STM image of the covalent dimer on a Ag(111) slab ( U =−0.6 V) with its carbon backbone. ( b ) High-resolution STM image of a dimer ( U =−0.57 V, I =0.1 nA). ( c ) STM image of an ordered dimer patch superimposed with the calculated dimer structure ( U =0.1 V, I =0.1 nA). All scale bars denote 10 Å. Full size image The combined insight from STM and DFT results reveals the covalent C−C linkage of ethynyl groups in a surface-assisted homo-coupling reaction. This process is illustrated in Fig. 1a . The generated hydrogen atoms are expected to recombinatively desorb as H 2 into the vacuum environment, following the previously established routes [20] , [29] , [30] . From the experimental fact that self-assembly of integral molecules readily occurs at low temperatures (cf. Fig. 2a ), we infer that molecular diffusion and rotation is not a limiting factor for the initial reaction steps. DFT investigation of the reaction pathway In our survey of possible pathways we started by hypothesizing the sophisticated model, elaborated on the basis of DFT calculations, for the reaction pathway of the Ullmann reaction of halobenzenes [31] , where the necessary cleavage of the C−X educt (X being a halogen unit) is expected to proceed readily in an isolated step on the surface, without introducing a major reaction barrier, whence the analysis can be restricted to the motion and interaction of chemisorbed C 6 H 5 units. Applied to the present system, we thus envisioned a precursor formation by the splitting-off of the hydrogen atoms of TEB molecules resulting in formally radical intermediates bound to the surface, followed by diffusion of these intermediates, and a covalent coupling reaction producing the dimer. Transition state calculations were carried out, and we found that in our case the initial C sp −H bond cleavage ( Fig. 4a ) implies a reaction barrier of 1.8 eV, being rather high compared with the overall energy barrier of 0.38 eV identified for the Ullmann reaction of C 6 H 5 units on Cu(111) that also proceeds at mild temperatures [31] . An alternative, putative mechanism via an adatom-related dehydrogenation ( Fig. 4b ) similar to the one proposed by King et al . [32] seems even more unlikely as it is associated with a reaction barrier of 1.9 eV. Moreover, there is no evidence for atomic steps playing a relevant role in the potential dehydrogenation according to the STM observations. 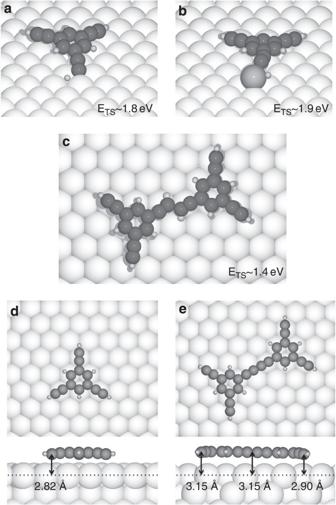Figure 4: DFT calculated possible transition states marking reaction barriers and adsorption geometries of the TEB monomer and the TEB dimer. The reaction barriers for (a) surface-catalysed and (b) adatom-catalysed dehydrogenation are remarkably higher than for (c) a direct covalent linking of two tautomerized TEB molecules. The energies of the transition states,ETS, are given with respect to the energy of an isolated molecule on the surface. (d) In the most favourable monomer adsorption configuration, the benzene ring is placed on a hollow site and the ethyne groups are centred over atop positions. (e) Only the right half of the covalently bonded dimer can adopt a geometry near to the optimal one displayed ind. The left half is forced to position the ethyne groups near to less favourable bridge sites. Accordingly, the dimer and particularly its left half resides at a larger height than the monomer. Figure 4: DFT calculated possible transition states marking reaction barriers and adsorption geometries of the TEB monomer and the TEB dimer. The reaction barriers for ( a ) surface-catalysed and ( b ) adatom-catalysed dehydrogenation are remarkably higher than for ( c ) a direct covalent linking of two tautomerized TEB molecules. The energies of the transition states, E TS , are given with respect to the energy of an isolated molecule on the surface. ( d ) In the most favourable monomer adsorption configuration, the benzene ring is placed on a hollow site and the ethyne groups are centred over atop positions. ( e ) Only the right half of the covalently bonded dimer can adopt a geometry near to the optimal one displayed in d . The left half is forced to position the ethyne groups near to less favourable bridge sites. Accordingly, the dimer and particularly its left half resides at a larger height than the monomer. Full size image Beyond previously established mechanisms we thus assessed a novel pathway implying a direct covalent bond formation, under the condition that the terminal alkyne group retains initially its integrity. Surface mobility of the constituents is not an issue, because self-assembly of regular TEB arrays readily occurs at T <200 K. Once two terminal alkyne moieties come in close proximity, a reaction intermediate can be achieved by invoking a connexion step producing a tautomerized dimer, followed by the splitting-off of the hydrogen atoms at a later stage. Our calculations suggest an appreciably lower reaction barrier of ~1.4 eV for the direct covalent linking of two TEB units via a nonlinear carbon chain ( Fig. 4c ). The necessary further step-by-step dissociations of the two hydrogen atoms and the reestablishment of the linear butadiyne bridge are almost spontaneous with barriers below ~0.15 eV. The reaction barrier of ~1.4 eV may be too high to match the experimental fact that dimerization readily takes place at T ~330 K. However, the employed reaction intermediate geometry was obtained by sticking closely to the covalent dimer coordinates. We expect to find transition states yielding smaller barriers by optimizing the tautomer geometry, for example, with respect to its conformation, the position of the H atoms or its registry with the substrate, which has not yet been done due to the related substantial computational effort. Even without further reduction, the barrier for the tautomerization pathway is already much smaller than the one associated with the covalent coupling of surface-stabilized cyclohexa- m -phenylene radicals on Ag(111), which is rate limited by the coupling step with a barrier of 1.8 eV [33] . Our barrier appreciably exceeds the 0.4 eV proposed for Ullmann coupling of phenyl on Cu(111) [31] (ref. 31 ), but this reaction is diffusion limited and thus for larger molecules much higher barriers interfere, as shown in ref. 33 . Our suggested reaction pathway involving a direct merging of two TEB units into the covalent dimer would explain why a higher flux is needed during the deposition to induce the reaction: as this is a second order reaction, a high coverage of molecules is needed to compete with the desorption of monomers, which are bonded to the surface by an adsorption energy of ~1.40 eV. Furthermore, our DFT calculations provide an explanation for the hierarchic character of the coupling reaction. The comparison of the monomer adsorption height (on average 2.93 Å above the Ag surface layer), with the dimer reveals a lifting of the latter by 0.19 Å. The most stable bonding geometries of the monomer and the dimer are compared in Fig. 4d and e where the adsorption heights of the alkyne groups are indicated. The monomer adsorbs symmetrically with the CH carbons of the alkyne group at a height of 2.82 Å. The dimer has no high-symmetry adsorption configuration with all alkyne groups adsorbed on equivalent surface sites. Only half the dimer adsorbs close to the geometry of the monomer, with the alkyne groups at a height of 2.90 Å. The other half of the molecule is adsorbed in a less favourable configuration explaining why this side of the molecule resides considerably further away from the surface. Supporting experimental evidence is provided by a comparison of the apparent height of monomer and dimer units in the same STM image ( Supplementary Fig. S3 ). TEB monomers exhibit a systematically lower value (0.87 Å) than the dimers (0.98 Å). Even though the apparent height values depend on the bias and cannot be compared with the geometric height directly, the bias independent tendency that dimers are systematically imaged higher than monomers is in agreement with theory. In addition, the slight asymmetric shape of the dimers is also consistent with the calculations. The increased adsorption height of the dimer compared to the monomer can be assigned to the mismatch between the dimer and Ag substrate. We note that the average adsorption height of the four favourable adsorption geometries for the monomer (cf. Supplementary Fig. S4 ) differ by 0.19 Å proving that small deviations of the most favourable adsorption geometry induce quite significant height changes. In addition, the covalently coupled alkynes may also have a negative effect on the interaction with the surface compared with the original terminal group. In any case, due to the lifting of the dimer compared with the monomer the catalytic effect of the surface is reduced after the first homo-coupling step, and any subsequent oligomerization implies increased energy barriers. This intriguing result indicates that the covalent coupling of the surface-confined terminal alkynes is sensitively influenced by the subtle details of the bonding geometry. It is suggested that this feature can be further explored to achieve site-selective linking of multitopic polyalkyne modules regulated by appropriate spacer groups at the respective terminal ethynyl groups. Such properties are sought for heterogeneous catalytic reactions or covalent engineering of hierarchic surface nano-architectures [34] . A comprehensive modelling of all possible pathways within the DFT framework is clearly beyond the scope of the present study, however, our present theoretical understanding strongly supports a new mechanism for the presented homo-coupling reaction on the Ag(111) surface. Generality of the on-surface homo-coupling To demonstrate the generality and further explore the noble metal surface-assisted alkyne homo-coupling reaction, we synthesized molecule 2 (1,3,5-tris-(4-ethynylphenyl)benzene; Ext-TEB; see Fig. 1b ). Depositing Ext-TEB molecules at low temperature (152 K) leads to the assembly of highly regular supramolecular domains ( Fig. 5a ) with flat-lying species and a packing scheme similar to that of TEB molecules. Following annealing of the covered surface to 300 K, again the characteristic dimers evolve, as shown in Fig. 5b , coexisting with unreacted precursor Ext-TEB species. Accordingly, the surface-assisted reaction is not outstripped by monomer desorption, which effect is ascribed to the stronger surface interaction. The imaging characteristics of the Ext-TEB dimers, in particular the resolution of the connecting waist and its overall length, can be explained on the same grounds as those of their TEB analogues. Hence, we conclude that the Ag(111) surface similarly promotes the Ext-TEB homo-coupling reaction, which process also obeys the hierarchic principle identified for the TEB species. 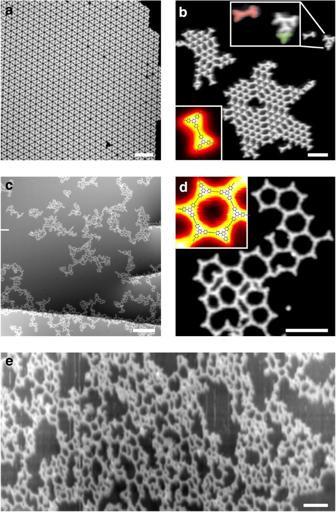Figure 5: STM topographic images of Ext-TEB molecules and reaction products on Ag(111). (a) Dense-packed phase formed by unreacted Ext-TEB molecules, deposited at a substrate temperature of 152 K. (b) Covalently bonded Ext-TEB dimers obtained by annealing at 300 K. The down-left inset shows a high-resolution image of a dimer superimposed with a HYPERCHEM calculated model. The upper inset magnifies an area with dimers (red) and monomers (green). (c) Large-scale image of covalent network patches, through annealing the sample to 400 K. (d) In the magnified area an open reticular structure from the merged ethynyl moieties prevails. The inset shows a single honeycomb nanopore superimposed with a HYPERCHEM calculated model. (e) STM overview image recorded at room temperature of a robust polymeric network structure obtained by irregular crosslinking at 520 K demonstrates the robustness of the structure at conditions relevant for later applications. The scale bars ina,b,dandedenote 50 Å, and inc250 Å. Figure 5: STM topographic images of Ext-TEB molecules and reaction products on Ag(111). ( a ) Dense-packed phase formed by unreacted Ext-TEB molecules, deposited at a substrate temperature of 152 K. ( b ) Covalently bonded Ext-TEB dimers obtained by annealing at 300 K. The down-left inset shows a high-resolution image of a dimer superimposed with a HYPERCHEM calculated model. The upper inset magnifies an area with dimers (red) and monomers (green). ( c ) Large-scale image of covalent network patches, through annealing the sample to 400 K. ( d ) In the magnified area an open reticular structure from the merged ethynyl moieties prevails. The inset shows a single honeycomb nanopore superimposed with a HYPERCHEM calculated model. ( e ) STM overview image recorded at room temperature of a robust polymeric network structure obtained by irregular crosslinking at 520 K demonstrates the robustness of the structure at conditions relevant for later applications. The scale bars in a , b , d and e denote 50 Å, and in c 250 Å. Full size image With the extended organic species, we managed to elaborate an even clearer picture of the polymerization reaction. A mild annealing treatment (400 K) leads to the formation of irregular, open-porous networks ( Fig. 5c ), that is, we again encounter a hierarchic reaction pathway. A closer inspection of the zoom-in (cf. Fig. 5d ) demonstrates the high level of purity achievable with our approach. Furthermore, it reveals that the covalently bonded architecture contains a series of features reflecting the pairwise connexion of the terminal ethynyl groups and a certain degree of molecular flexibility. The six-membered oligomeric cyclic units represent the ideal product of a convergent homo-coupling reaction with straight C−C connexions between the Ext-TEB modules. The inset shows a magnified image of the associated honeycomb unit, and a corresponding HYPERCHEM model that nicely fits the STM data. By contrast, the additional five- and seven-fold cyclic structures imply distortions of the molecular modules [27] , [28] , [35] . In addition, some features are visible where three molecular terminations join together, which can be of different origin including covalent connexions differing from the intended butadiyne bridges as further discussed in the Supplementary Information ( Supplementary Fig. S5 ). Next, we demonstrate the formation of extended 2D polymeric networks using the surface-assisted coupling protocol. The STM image in Fig. 5e reveals that a coherently reticulated layer structure decorating the entire silver substrate can be readily achieved with the thermal treatment of high Ext-TEB surface concentrations. Importantly, this reaction product is robust and its stable character becomes obvious in STM data recorded at room temperature. The layer formation reflects an irregular crosslinking process. In this sample the deviations from the ideal linear butadiyne bridges are more frequent than in the previous sample ( Fig. 5d ). We attribute this to the fact that before the thermal treatment a higher molecular coverage was present and the maximum annealing temperature was 520 K. The combination of both probably gives rise to more types of covalent connexions differing from the intended one. Because the lateral C−C linkages between the Ext-TEB modules are stronger than the surface bonding of individual units, the layer represents a covalent nanomembrane that can be potentially used in further processing steps and applications, similar to related 2D sheets [9] , [10] , [36] , [37] . Complementary X-ray photoelectron spectroscopy evidence Finally, the claimed covalent bond formation is substantiated by complementary X-ray photoelectron spectroscopy (XPS) measurements. We investigated a sample prepared under comparable conditions as the one showing the reticulated Ext-TEB network, that is, evaporation of Ext-TEB onto the Ag(111) surface at 315 K followed by mild annealing to 400 K. In the C1s region ( Fig. 6a ) only a single discernable peak is present at a binding energy of 284.9 eV resulting from a superposition of several carbon species with binding energies differing by less than the energy resolution. Owing to the overlapping of the signals of the chemically slightly different carbon species, the experimental profile was fitted with only two general Voigt peaks that do not represent a distinct carbon species each. As a typical binding energy for methylacetylide on Ag(111) is 283.7 eV [38] (ref.38), the absence of such a low-energy shoulder already indicates the absence of organometallic bonding in our sample. Further support for the covalent character is provided by a DFT-based simulation of XPS line shapes ( Fig. 6b ) of a covalent TEB dimer ( Fig. 6c ) and an organometallic dimer ( Fig. 6d ). In this simulation we used the smaller TEB species instead of the larger Ext-TEB due to computation time limitations. The geometries of the respective adsorbates were optimized on the Ag(111) slab and then the C1s core-level shifts were calculated for each carbon atom with reference to an arbitrarily chosen atom (cf. Fig. 6c and Supplementary Fig. S6 ). Then for each carbon atom a Voigt peak with a shape expected for our experimental resolution of ~0.6 eV was generated and the peaks were superposed taking into account the relative energy shifts. The resulting simulated signals were placed on the same energy axis as the experimental spectra in order to facilitate comparison ( Fig. 6a ). Consistent with the literature our simulation of the organometallic dimer (red dashed line) shows a low binding energy shoulder originating from the ethynyl groups interacting with the Ag atom. In the case of an Ext-TEB network where most of the ethynyl groups are coordinated to a silver atom, approximately the same relative intensity of this shoulder is expected. Thus, the low-energy component should be clearly discernable with our experimental resolution. However, no such component is visible in the experimental data. Therefore, the XPS analysis strongly opposes to a potential organometallic binding mechanism behind the formation of the 2D polymeric network in agreement with our combined STM/DFT analysis. 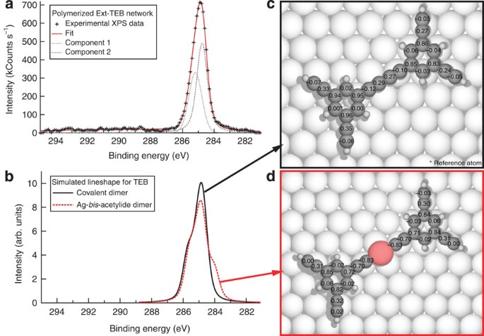Figure 6: XPS data of polymerized Ext-TEB network and DFT-based simulated line shapes calculated from covalent and organometallic dimers. (a) Experimental XPS data of the C1s region of a sample with a submonolayer coverage of Ext-TEB after annealing to 400 K. The experimental spectrum (crosses) show a single peak centred at 284.9 eV. (b) DFT-based simulation of the XPS line shape of the covalent (black solid line) and the organometallic (red dashed line) TEB dimer expected for an experimental resolution of ~0.6 eV. (c,d) Top view of the DFT-optimized adsorption geometry of a covalent and an organometallic TEB dimer, respectively. The C1s core-level shifts relative to the reference atom are superimposed on each carbon atom. The Ag atom incorporated into the organometallic dimer is highlighted in red ind. arb., arbitrary. Figure 6: XPS data of polymerized Ext-TEB network and DFT-based simulated line shapes calculated from covalent and organometallic dimers. ( a ) Experimental XPS data of the C1s region of a sample with a submonolayer coverage of Ext-TEB after annealing to 400 K. The experimental spectrum (crosses) show a single peak centred at 284.9 eV. ( b ) DFT-based simulation of the XPS line shape of the covalent (black solid line) and the organometallic (red dashed line) TEB dimer expected for an experimental resolution of ~0.6 eV. ( c , d ) Top view of the DFT-optimized adsorption geometry of a covalent and an organometallic TEB dimer, respectively. The C1s core-level shifts relative to the reference atom are superimposed on each carbon atom. The Ag atom incorporated into the organometallic dimer is highlighted in red in d . arb., arbitrary. Full size image In solution chemistry, the formation of π-alkyne-silver complexes is an initial step on the way to acetylides, that is, between silver cations and terminal C−H bond a nonlinear two-electron, three-centre bond is formed (for a thorough discussion cf. refs 22 , 23 ). With the surface confinement the planar adsorption of the presently investigated organic species entails a natural proximity between the Ag surface atoms and the ethynyl group. This geometry profoundly influences the chemical nature of the terminal alkyne. From the mild temperatures at which the homo-coupling takes place, it can be concluded that the very presence of the Ag(111) substrate indeed supplies a catalytic template. The hierarchic steps in which the reaction proceeds demonstrate how sensitive the alkyne C−H activation and reactivity responds to subtle changes of the local environment. Moreover, with the reaction pathway being established via a tautomerized intermediate, there is no need to a priori invoke an organometallic reaction intermediate, that is, there is a formal similarity with the envisioned mechanism in silver acetylide formation in the presence of a base [23] , being at variance with related processes mediated by transient attachment of copper ions at the ethynyl group [32] . It is also interesting to note that it was impossible to induce covalent bonding of acetylene molecules on an oxide surface by the presence of single silver atoms [39] . To conclude, we introduced a novel heterogeneous catalytic synthesis protocol for the surface-confined coupling of terminal alkyne species at a smooth noble metal substrate. Our systematic STM measurements and DFT calculations demonstrate covalent C−C bonding and 2D polymerization through homo-coupling reactions in a surface-assisted synthesis proceeding in vacuum under mild conditions without generation of spurious by-products. With multifunctional species (for example, the presently employed tritopic compounds) product formation is affected and tunable by hierarchic reaction pathways, reflecting the modified surface interaction of reaction intermediates. It is suggested that terminal alkyne building blocks can be in general covalently linked on suitable noble metal surfaces to create novel molecular compounds, low-dimensional superstructures or coherently reticulated polymeric layers. This provides a new synthesis route towards conjugated molecular nanosystems and networks, providing potential for the fabrication of regular 1D scaffolds, such as carbyne [40] , [41] , 2D polymers, such as graphyne or graphdiyne [6] , [42] , and similar hydrocarbon membranes. We furthermore envision the use of nanostructured interfaces and noble metal nanoparticles as catalytic materials and reaction templates under vacuum or other conditions. Synthesis The 1,3,5-triethynyl arenes ( 1 ) and ( 2 ) ( Supplementary Fig. 7 ) were obtained according published procedure [43] by coupling of aryl bromides ( 3 ) and ( 4 ) ( Supplementary Fig. 7 ) and trimethylsilylacetylene in the presence of the catalytic system copper(I)iodide, bis(triphenylphosphine)palladium(II) dichloride (Pd(PPh 3 ) 2 Cl 2 -CuI)) and secondary amine as solvent and base. The resulting silyl intermediates ( 5 ) and ( 6 ) ( Supplementary Fig. 7 ) were hydrolysed to yield 86% and 75% of 1,3,5-triethynylbenzene ( 1 ) and 1,3,5-tris-(4-ethynylphenyl)benzene ( 2 ), respectively. Sample preparation The experiments were carried out in an UHV apparatus with a base pressure of less than 2 × 10 −10 mbar. The Ag(111) single crystal surface was prepared by repeated cycles of Ar + ion sputtering, followed by annealing to 740 K. Both compounds were sublimated by organic molecular beam epitaxy (OMBE) from a quartz glass crucible inside a Knudsen cell. For Ext-TEB molecules, a purified powder has been used; the sublimation temperature T OMBE was in the ~420–450 K range. For TEB molecules we had to use a non-purified powder, introducing a small concentration of contaminations on the surface. The related impurities do not interfere in the surface processes, as evidenced by the self-assembly of the pure species (cf. Fig. 2a ). In UHV the room temperature vapour pressure of TEB is finite. As a result the molecular flux obtained at a specific T OMBE reduces with time after filling of the crucible. For the sample shown in Fig. 2b T OMBE was room temperature. The higher flux used for subsequent experiments was achieved by a new refill of TEB molecules into the crucible, that is, it did not imply increased evaporation temperatures. To avoid polymerization for TEB molecules in the crucible, the sublimation temperature was strictly kept below 370 K for all preparations. Sublimating TEB molecules ( T OMBE <370 K) onto the cold Ag(111) substrate held at 170 K, no signature of covalent reaction was found. After the preparation, the sample was cooled down and transferred into our home-made Besocke-type STM [44] , where data were recorded with a chemically etched tungsten tip at 5.5 K (unless mentioned otherwise). The bias for tunnelling current is applied to the sample. If not stated otherwise, typical tunnelling condition were U =−1 V and I =0.1 nA. DFT calculations Periodic DFT calculations were carried out with the VASP code [45] , with ion-core interactions described by the projected augmented wave method [46] , [47] . A variant of the van der Waals density functional [48] was used, with the exchange replaced by an optimized form of the Becke 86 exchange functional [49] . The plane waves were expanded to a cutoff of 500 eV and the Γ-point was used to sample the first Brillouin zone. A p(7 × 7) and p(10 × 9) unit cell were used in the calculations of TEB monomer and dimer, respectively. The Ag(111) surface was modelled by four layered slabs. All structures were relaxed until the forces on the atoms in the adsorbate and the two outermost layers of the slab were smaller than 0.01 eV Å −1 . STM images were calculated using the Tersoff–Hamann approximation [50] , as implemented by Lorente and Persson [51] . Energy barriers were obtained by transition state calculations following the approach described in ref. 52 using a combination of the climbing image nudged elastic band [53] (CI-NEB) and Dimer [54] , [55] methods. In short, CI-NEB was used to find an initial estimate of the transition state. The estimate was then used to generate the input (central image and dimer) in the Dimer method. Structural optimization of the dimer was performed until the forces acting on the atoms in the central images were smaller than 0.04 eV Å −1 . Simulated core-level shifts were obtained by comparing total energy differences between core-ionized and ground state systems. The total energies of core-ionized systems were computed by using a core-ionized projected augmented wave potential for the core-ionized atom as described by Köhler and Kresse [56] . Hence, a separate calculation was carried out for every atom for which the core-level shift was computed. In this way, not only the local electrostatic potential of the atoms, but also screening of the core-hole in the final state is taken into account when simulating the core-level shifts. Similar calculations yielded reasonable results and proved to be helpful for the understanding of bonding properties in surface anchoring of organic species [57] and on-surface molecular architectures [58] . X-ray photoelectron spectroscopy The XPS measurements were carried out at the HE-SGM monochromator dipole magnet beam line at the BESSY II synchrotron radiation source in Berlin, which provides light with a linear polarization of 90%. Samples were prepared in situ in ultrahigh vacuum, employing the protocols described above. Electrons were collected using a Scienta R3000 electron energy analyser in perpendicular emission mode. HYPERCHEM calculations The HYPERCHEM software (HYPERCHEM, Hypercube Inc., Gainesville, FL) was used to calculate the models of the Ext-TEB dimer and hexagon in Fig. 5 . Both geometries were optimized with semi-empirical methods using the AM1 model. How to cite this article: Zhang, Y.Q. et al . Homo-coupling of terminal alkynes on a noble metal surface. Nat. Commun. 3:1286 doi: 10.1038/ncomms2291 (2012).